A model of parity-dependent immunity to placental malaria Plasmodium falciparum placental infection during pregnancy is harmful for both mother and child. Protection from placental infection is parity-dependent, that is, acquired over consecutive pregnancies. However, the infection status of the placenta can only be assessed at delivery. Here, to better understand the mechanism underlying this parity-dependence, we fitted a model linking malaria dynamics within the general population to observed placental histology. Our results suggest that immunity resulting in less prolonged infection is a greater determinant of the parity-specific patterns than immunity that prevents placental sequestration. Our results also suggest the time when maternal blood first flows into the placenta is a high-risk period. Therefore, preventative strategies implementable before or early in pregnancy, such as insecticide-treated net usage in women of child-bearing age or any future vaccine, could substantially reduce the number of women who experience placental infection. Each year an estimated 55 million pregnancies occur within areas of stable Plasmodium falciparum transmission [1] . Acquiring malaria in pregnancy (MiP) can have severe adverse consequences for both mother and child. MiP is a major contributing cause of maternal anaemia, with an estimated population attributable fraction of 26% of all cases of severe anaemia in pregnant women in sub-Saharan Africa [2] , [3] . MiP also markedly increases the likelihood of low birth weight (LBW), due to both pre-term delivery and foetal growth restriction [4] , [5] , which leads to a high risk of neonatal and infant mortality and is associated with a range of adverse developmental outcomes during infancy and later in life [2] . The adverse consequences associated with P. falciparum infection affect women in a distinctive, parity-dependent manner, with primigravidae at much higher risk of infection than multigravidae, and consequently of anaemia and LBW deliveries. This pattern has been found to be independent of any age-dependent effects and is thought to occur as the result of placental infection, whereby infected erythrocytes (IEs) accumulate within the maternal intervillous space [2] , [6] , [7] , [8] . Such sequestration only takes place from late in the third month of gestation onwards [9] , as the placenta needs first to develop to the point where maternal blood begins flowing into the intervillous space, which is thought to take place by the end of the 12th week of gestation [10] , [11] . Once the placenta has reached this stage of development, IEs begin to adhere to receptors on the surface of placental villi mediating their accumulation in the intervillous space [12] . This accumulation of parasites within the maternal vasculature of the placenta, when in sufficiently large numbers, triggers an infiltration of maternal immune cells [13] , [14] . This in turn can lead to the upregulation of inflammatory cytokines and to large-scale fibrin deposits within the placenta [6] , [15] . This inflammatory immune response, though possibly effective at limiting parasite replication, may be less efficient at clearing parasitaemia, producing a prolonged chronic infection [7] . It is this chronic stage of placental infection that has been most strongly associated with both severe anaemia and foetal growth restriction [10] , [14] , [16] . In contrast, the acute stage of infection before immune cell infiltration has been more closely associated with pre-term births, particularly among symptomatic women [4] , [6] . The decreasing prevalence of placental infection and decreasing severity of the associated adverse consequences during pregnancy with increasing parity, independent of the mother’s age, suggests that women acquire protection from P. falciparum MiP with successive pregnancies [17] , [18] . Evidence for parity-dependent immunity also comes from the finding that antibodies capable of inhibiting adhesion to CSA are acquired over successive pregnancies and that these antibodies are associated with increased birth weight and, in some cases, increased maternal haemoglobin level [6] , [19] , [20] . However, to date, the effects of parity-dependent immunity upon the dynamics of placental malaria, in terms of the likelihood of IE sequestration following infection and the duration of placental infection, have not been systematically quantified. At delivery, histological analysis of placental tissue remains the most accurate indicator of ongoing placental sequestration and can also provide an indication of the stage of infection through assessment of the histological changes, which have occurred within the placenta [21] , [22] . However, such analysis can only be conducted at delivery. Throughout pregnancy, the prevalence of placental infection can only be assessed indirectly in samples from peripheral blood. Peripheral infection at delivery is usually a good indicator of an ongoing placental infection, however, such measures generally underestimate the prevalence of sequestration and woman with placental infection often remain asymptomatic [21] . As a result, many placental infections are likely to go undetected until delivery and it is not possible to accurately assess the timing and duration of infection during pregnancy. Here, we develop a mathematical model of placental malaria for P. falciparum infection, exploring a range of different mechanisms for the development of parity-dependent immunity. We use the model to better understand the relationship between transmission intensity and the age- and parity-dependent risk of placental malaria in areas of moderate to high transmission intensity. We use placental histology data from two different transmission settings to estimate the duration of the four histologically relevant stages of placental infection. We also investigate the ways in which the development of immunity as a function of placental infection in previous pregnancies can explain the observed histology results across different parity strata. Using these estimated parameters we then derive a relationship between the prevalence of placental infection by parity, stage of infection (past or active, with active infection further divided into acute or chronic stages) and gestational age and the transmission intensity within a given setting and discuss the possible implications these results have for both the medium- and long-term effects of treatment and prevention strategies. 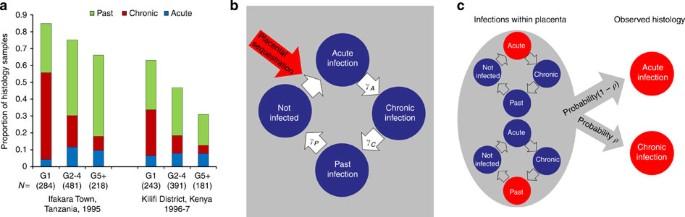Figure 1: Histology data and model of placental infection. (a) The proportion of histology samples in each gravidity category in each study, which were classified as acute, chronic and past infections. The number of samples in each category is displayed below each gravidity category label in parentheses. (b) When placental sequestration occurs this results in an ‘acute infection’, the infection then passes through the remaining stages of placental infection according to the stage-specific rates of progression until, if the pregnancy has yet to reach delivery, all evidence of sequestration is fully cleared. (c) When infection within the placenta consists of a combination of a recent acute infection and pigment from a previous infection, the observed histology depends upon whether the earlier infection has left behind ‘substantial pigment’ (with probabilityP) in which case the overall result would be defined as ‘chronic’ infection. Otherwise the result would be classed as ‘acute’ infection. Mechanisms of parity-dependent immunity Figure 1a shows the proportion of histology samples that were graded as acute, chronic and past infection stratified by gravidity from two surveys of the placentas of women residing in endemic areas—Kilifi, Kenya [23] and Ifakara Town, Tanzania [16] . A clear pattern is observed in both settings with a higher proportion of chronic infections in primigravidae. Using a mathematical model of the progression of placental infection through each of the histological stages ( Fig. 1b ), we explored which immune mechanisms could explain this pattern. The different models of immunity considered are detailed in Table 1 . In total, four mechanisms for parity-dependent immunity were tested. First, we assumed that immunity would act by reducing the susceptibility to placental infection in subsequent pregnancies; second, we assumed that immunity would speed the transition from the acute stage to the chronic stage; third, we assumed that immunity would speed the transition from the chronic stage to the past stage; and fourth, we assumed that immunity would speed the transition from the past stage to no infection. Our third model, namely an increase in the rate at which chronic infection is cleared, provided the best fit of the single mechanism models to the observed histology data ( Supplementary Table S3 ). Overall, when allowing parity-dependent immunity to act through more than one mechanism, the best fitting model was one where the faster clearance of chronic infection was coupled with sequestration-blocking immunity ( Fig. 2a , Supplementary Table S3 ). A better fit to the data could not be achieved by the addition of parity-dependent clearance of either the acute or the past stage of infection. As a result, we chose the model combining sequestration blocking and a faster clearance of chronic infection as our final model with which to conduct the remainder of our analysis. Figure 1: Histology data and model of placental infection. ( a ) The proportion of histology samples in each gravidity category in each study, which were classified as acute, chronic and past infections. The number of samples in each category is displayed below each gravidity category label in parentheses. ( b ) When placental sequestration occurs this results in an ‘acute infection’, the infection then passes through the remaining stages of placental infection according to the stage-specific rates of progression until, if the pregnancy has yet to reach delivery, all evidence of sequestration is fully cleared. ( c ) When infection within the placenta consists of a combination of a recent acute infection and pigment from a previous infection, the observed histology depends upon whether the earlier infection has left behind ‘substantial pigment’ (with probability P ) in which case the overall result would be defined as ‘chronic’ infection. Otherwise the result would be classed as ‘acute’ infection. Full size image Table 1 The different models of immunity investigated in the model. 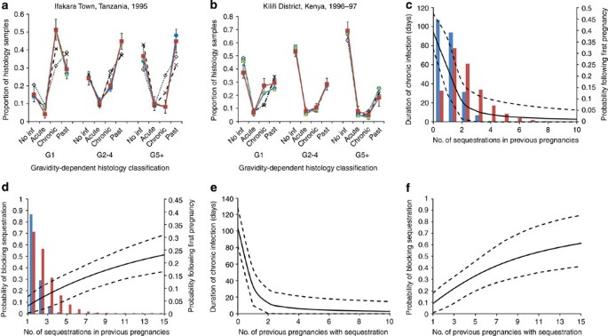Figure 2: Final fitted models and immunity functions. (a,b) Show the fit of the model to the placental histology data from Ifakara and Kilifi, respectively. Observed data are represented by the red lines and squares, error bars are 95% binomial confidence intervals based upon the fact that, when assuming a multinomial distribution, each individual point follows a binomial distribution. Blue lines and circles show the posterior mean of the proportion of samples in each category according to the final infection-dependent model and green dashed lines and triangles show the equivalent for the final infected-pregnancy-dependent model. For comparison, lines showing the equivalent values for the model assuming no parity-dependent immunity (dotted black line with open diamonds) and the infected-pregnancy-dependent model with only sequestration-blocking immunity (dashed black lines with crosses) have also been plotted. (c) Shows how the duration of chronic infection decreases and (d) the extent to which placental infection is prevented with increased exposure to placental infection in prior pregnancies for the ‘infection-dependent’ immunity assumptions and (e,f) the equivalent figures for the ‘infected-pregnancy-dependent’ assumption. For the infection-dependent figures the distributions of the number of placental infections experienced throughout first pregnancies in Ifakara (red bars) and Kilifi (blue bars) are also shown. Full size table Figure 2: Final fitted models and immunity functions. ( a , b ) Show the fit of the model to the placental histology data from Ifakara and Kilifi, respectively. Observed data are represented by the red lines and squares, error bars are 95% binomial confidence intervals based upon the fact that, when assuming a multinomial distribution, each individual point follows a binomial distribution. Blue lines and circles show the posterior mean of the proportion of samples in each category according to the final infection-dependent model and green dashed lines and triangles show the equivalent for the final infected-pregnancy-dependent model. For comparison, lines showing the equivalent values for the model assuming no parity-dependent immunity (dotted black line with open diamonds) and the infected-pregnancy-dependent model with only sequestration-blocking immunity (dashed black lines with crosses) have also been plotted. ( c ) Shows how the duration of chronic infection decreases and ( d ) the extent to which placental infection is prevented with increased exposure to placental infection in prior pregnancies for the ‘infection-dependent’ immunity assumptions and ( e , f ) the equivalent figures for the ‘infected-pregnancy-dependent’ assumption. For the infection-dependent figures the distributions of the number of placental infections experienced throughout first pregnancies in Ifakara (red bars) and Kilifi (blue bars) are also shown. Full size image We also explored two ways in which previous infection could determine the degree of immunity ( Table 1 ). First (which we term ‘infection-dependent immunity’), we assumed that the level of immunity was a function of the number of placental infections previously experienced (allowing for multiple infections in a single pregnancy). Second (which we term ‘infected-pregnancy-dependent immunity’) we assumed that the level of immunity was a function of the number of pregnancies in which placental infection had occurred. It was not possible, however, to differentiate between these models with both immunity assumptions providing a good but near identical fit to the two data sets ( Fig. 2a ). From both models we estimate a mean duration of the chronic stage of infection in primigravidae of around 100 days (see Table 2 ), if left untreated. This duration is estimated to decrease sharply with exposure in previous pregnancies ( Fig. 2c ). In contrast, our estimates suggest that sequestration-blocking immunity develops relatively slowly and appears to saturate with ∼ 50% of placental infections prevented ( Fig. 2d ). We further estimate a 50-day mean duration of acute stage infection and a rate of transition through the ‘past infection’ stage (the stage where all parasites have been cleared and only pigment remains), which would appear to suggest that, by delivery and in the absence of treatment, the pigment associated with placental sequestration is rarely fully cleared ( Table 2 ). Our estimates of the proportion of infections, which leave ‘significant’ pigment following the clearance of parasites, were not very precise but, for both final models, the 95% credible intervals fall entirely below 0.8. This appears to indicate that, as the definition of acute infection proposed by Ismail et al . [23] would suggest (see Materials and Methods), a proportion of histology samples diagnosed as acute infections could be expected additionally to contain some evidence of previous infection in the form of ‘minimal pigment’. Although the mean duration of acute infection changed very slightly, the main results of our analysis were insensitive to the different assumed durations between infection and sequestration within the placenta (see Supplementary Table S5 ). We also found that decreasing the proportion of infections, which have the ability to sequester within the placenta, had little effect upon our estimated model parameters apart from inflating our fitted EIR in each setting and progressively worsened the fit of the model to the data ( Supplementary Table S4 ). Table 2 Fitted parameters for the two final placental malaria models. 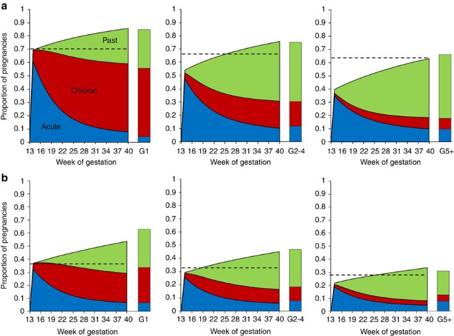Figure 3: Estimates of the prevalence of each histological stage by week of gestation. (a) Shows the posterior mean estimated prevalence of each stage of sequestration during each week of gestation for the Ifakara transmission setting. (b) Shows the equivalent figure for the Kilifi transmission setting. In each figure, blue areas show the prevalence of acute stage infection, red the prevalence of chronic stage infection and green the prevalence of past stage infection. In each figure, the left chart shows the estimate for primigravidae, the central chart shows gravidities 2–4 and the right chart shows gravidities 5 and above. The observed data for each gravidity category and transmission setting, as shown in Fig. 1, is presented as a column beside the appropriate chart. The age-adjusted prevalence of parasitaemia for each category is presented as a dashed black line. Full size table The prevalence of placental infection throughout gestation Figure 3 shows the estimated prevalence of each stage of infection as a function of gestational duration. Our estimates suggest that pregnant women are most at risk of placental malaria immediately after the placenta becomes susceptible to parasitization, which occurs at the end of the third month of gestation in our baseline model. According to our model assumptions, this is the stage where any circulating parasites are first able to sequester (in the absence of sequestration-blocking immunity). As a result, in the modelled primigravidae, the incidence of placental sequestration at this stage of gestation is equivalent to the age-adjusted prevalence of parasitaemia in the general population. Following this key high-risk period, the incidence of new sequestration events falls back to the incidence of infection in the general population. Therefore, although the proportion of women with any stage of placental infection steadily rises throughout gestation, the proportion with active (acute or chronic) placental infection is predicted to decline. We estimate that, as a result of this pattern of infection throughout pregnancy, only 30% ( Fig. 4a ; green areas) of the time spent with infection during first pregnancies can be attributed to infection occuring after the placenta becomes susceptible and only 50% ( Fig. 4b ; green areas) to infection occuring at any time during the pregnancy. Conversely, taking into account multiple infections, in all but the most intense transmission settings, the majority of time spent with placental infection is due to infections acquired before the placenta first becomes susceptible, with the majority of these infections acquired before the beginning of pregnancy. Figure 3: Estimates of the prevalence of each histological stage by week of gestation. ( a ) Shows the posterior mean estimated prevalence of each stage of sequestration during each week of gestation for the Ifakara transmission setting. ( b ) Shows the equivalent figure for the Kilifi transmission setting. In each figure, blue areas show the prevalence of acute stage infection, red the prevalence of chronic stage infection and green the prevalence of past stage infection. In each figure, the left chart shows the estimate for primigravidae, the central chart shows gravidities 2–4 and the right chart shows gravidities 5 and above. The observed data for each gravidity category and transmission setting, as shown in Fig. 1, is presented as a column beside the appropriate chart. The age-adjusted prevalence of parasitaemia for each category is presented as a dashed black line. 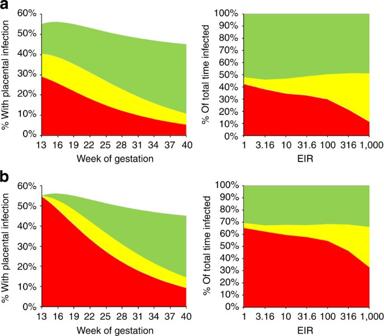Figure 4: The impact of infection before and early during first pregnancy. (a) Shows the time spent with placental infection during first pregnancy caused by infections acquired before (that is, <0 weeks gestation-red areas) and during (that is,⩾0 weeks gestation-green areas) pregnancy, yellow areas show time spent with multiple placental infections caused by infection acquired both before and during pregnancy. (b) Shows the equivalent figure but partioning the prevalence of placental infection according to whether placental infection is due to infection acquired before the placenta first becomes susceptible to infection (that is, <12 weeks gestation), with yellow areas showing time spent with placental infections caused by infection acquired both before and during this point in gestation. In both cases, the chart on the left shows how infections acquired at the different stages change with gestational time in an area with EIR=100 and the chart on the right shows the proportion of the total time spent with placental infection by EIR. Full size image Figure 4: The impact of infection before and early during first pregnancy. ( a ) Shows the time spent with placental infection during first pregnancy caused by infections acquired before (that is, <0 weeks gestation-red areas) and during (that is, ⩾ 0 weeks gestation-green areas) pregnancy, yellow areas show time spent with multiple placental infections caused by infection acquired both before and during pregnancy. ( b ) Shows the equivalent figure but partioning the prevalence of placental infection according to whether placental infection is due to infection acquired before the placenta first becomes susceptible to infection (that is, <12 weeks gestation), with yellow areas showing time spent with placental infections caused by infection acquired both before and during this point in gestation. In both cases, the chart on the left shows how infections acquired at the different stages change with gestational time in an area with EIR=100 and the chart on the right shows the proportion of the total time spent with placental infection by EIR. Full size image A similar qualitative pattern is also estimated for women of higher parity, although, because of the effects of parity-dependent immunity, a proportion of infections do not sequester meaning the incidence peaks below the age-adjusted prevalence. The prevalence of infection then falls much more sharply than in primigravidae as these women progress more rapidly through the chronic stage of infection. Moreover, as they are drawn from an older cohort, they experience a lower age-adjusted prevalence and incidence of infection outside of pregnancy. This results in women of higher parity experiencing both a lower initial peak in prevalence and a lower incidence of placental sequestration throughout the remainder of the pregnancy. The effects of parity-dependent immunity also mean that the proportion of women with chronic infection, both at delivery and throughout gestation, is predicted to decrease markedly in women of higher parity. In contrast, as the number of acute infections is essentially a measure of the number of placentas, which have been recently parasitized, and there was no evidence of parity-dependent immunity acting on this stage of infection, the proportion of women with acute infection at delivery stays relatively constant across parity classes ( Fig. 5a ). 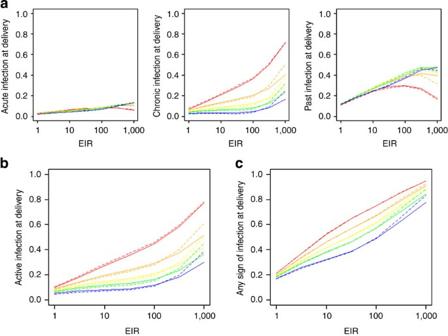Figure 5: Prevalence of placental sequestration at delivery by EIR. In each red lines show G1 pregnancies, orange lines G2, yellow lines G3, green lines G4 and blue lines G5+. Solid lines show the infection-dependent immunity and dashed lines show infected-pregnancy-dependent immunity. (a) Shows the posterior mean prevalence of acute, chronic, and past infection. (b) The prevalence of active infection (acute or chronic) at delivery and (c) the prevalence of any sign of infection (acute, chronic or past) at delivery. Figure 5: Prevalence of placental sequestration at delivery by EIR. In each red lines show G1 pregnancies, orange lines G2, yellow lines G3, green lines G4 and blue lines G5+. Solid lines show the infection-dependent immunity and dashed lines show infected-pregnancy-dependent immunity. ( a ) Shows the posterior mean prevalence of acute, chronic, and past infection. ( b ) The prevalence of active infection (acute or chronic) at delivery and ( c ) the prevalence of any sign of infection (acute, chronic or past) at delivery. Full size image Transmission intensity and placental infection prevalence The proportion of women of any parity with evidence of placental sequestration increases steadily with increasing EIR ( Fig. 5c ). However, at EIRs between around 3 and 30 the proportion of women with active infection at delivery plateaus at higher parities. This is because, at these levels of transmission, increases in exposure to infectious bites are predicted to be offset by the faster clearance of infection following the development of parity-dependent immunity ( Fig. 5b ). In contrast, the prevalence of both active infection and placentas with any evidence of infection at delivery increases rapidly in all gravidities as the EIR passes 100. At this high level of transmission the incidence of infection throughout gestation overwhelms the maximum level of immunity estimated by the model. Effect of the timing of IPTp To investigate the timings at which preventative treatment may be most important, the effects of a drug, which clears any placental infection and provides protection for a mean of 20 days given at either 10, 20 or 30 weeks, was calculated for different EIRs. Our results indicate that the observed effect of a single dose of preventative therapy on the prevalence of active (acute or chronic) placental infection at delivery will be greatest if the drug is adminstered later in pregnancy ( Fig. 6a ). However, the overall effectiveness of IPTp (if measured by the proportion of women who ever experience chronic infection) will be greatest when the dose is adminstered earlier in pregnancy. Moreover, our model suggests that when the first dose is adminstered after foetal quickening (around 18–20 weeks in first pregnancies and 15–17 weeks in subsequent pregnancies [24] ), in accordance with current guidelines, IPTp may have little impact on the number of women who ever experience placental infection. This is because most placental infections are predicted to occur before this point. In contrast, our model predicts that the same dose of preventative therapy administered at 10 weeks would prevent a larger number of chronic infections and would substantially reduce the number of women who ever experience placental sequestration. For the scenarios tested, early adminstration of a single dose of preventative therapy would outperform the current recommended double dose strategy in all but the highest transmission intensity settings ( Fig. 6b ). 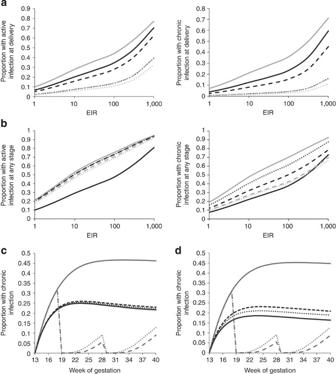Figure 6: The potential impact of preventative therapy. (a) Shows both the prevalence of active (acute or chronic) and the prevalence of chronic infection in primigravidae at delivery. (b) Shows the total proportion of primigravidae experiencing placental infection of this type at any stage of their pregnancy. In both (a,b), grey solid lines show estimates in the absence of any intervention, black lines show estimates when a single dose of preventative therapy (resulting in a Gamma-distributed period of prophylaxisP∼Γ(4,5), with a mean of 20 days) is adminstered at 10 (solid lines), 20 (dashed lines) and 30 (dotted lines) weeks gestation, grey dashed lines show estimates when IPT with the same effect is adminstered at 20 and 20 weeks and grey dotted lines show the same two-dose regimen with a mean period of prophylaxis of 30 days following each dose,P∼Γ(5,6). Results shown are posterior mean estimates from the infection-dependent final model. In (c,d), grey lines show the predicted prevalence of chronic infection in primigravidae in the absence of preventative therapy for the Ifakara transmission setting (solid grey lines), the scenario where IPTp is admistered at 18 and 28 weeks and prophylaxis lasts an average of 30 days,P∼Γ(5,6), (dashed lines) and an average of 15 days,P∼Γ(3,5), (dotted lines). Black lines show the prevalence of chronic infection in the same cohorts during their second pregnancy when IPTp is not adminstered. (c) Shows the scenario where immunity is infected-pregnancy-dependent and (d) where immunity is infection-dependent. In all figures ‘chronic infection’ refers only to chronic infections, which have moved through an acute stage, rather than chronic infections, which are a mixture of an acute and past infection. Figure 6: The potential impact of preventative therapy. ( a ) Shows both the prevalence of active (acute or chronic) and the prevalence of chronic infection in primigravidae at delivery. ( b ) Shows the total proportion of primigravidae experiencing placental infection of this type at any stage of their pregnancy. In both ( a , b ), grey solid lines show estimates in the absence of any intervention, black lines show estimates when a single dose of preventative therapy (resulting in a Gamma-distributed period of prophylaxis P ∼ Γ(4,5), with a mean of 20 days) is adminstered at 10 (solid lines), 20 (dashed lines) and 30 (dotted lines) weeks gestation, grey dashed lines show estimates when IPT with the same effect is adminstered at 20 and 20 weeks and grey dotted lines show the same two-dose regimen with a mean period of prophylaxis of 30 days following each dose, P ∼ Γ(5,6). Results shown are posterior mean estimates from the infection-dependent final model. In ( c , d ), grey lines show the predicted prevalence of chronic infection in primigravidae in the absence of preventative therapy for the Ifakara transmission setting (solid grey lines), the scenario where IPTp is admistered at 18 and 28 weeks and prophylaxis lasts an average of 30 days, P ∼ Γ(5,6), (dashed lines) and an average of 15 days, P ∼ Γ(3,5), (dotted lines). Black lines show the prevalence of chronic infection in the same cohorts during their second pregnancy when IPTp is not adminstered. ( c ) Shows the scenario where immunity is infected-pregnancy-dependent and ( d ) where immunity is infection-dependent. In all figures ‘chronic infection’ refers only to chronic infections, which have moved through an acute stage, rather than chronic infections, which are a mixture of an acute and past infection. Full size image Implications of assumptions about infection and immunity As our model predicts that the first dose would be administered after the majority of first infections during pregnancy, IPT would have little effect upon the acquision of any ‘infected-pregnancy-dependent’ immunity ( Fig. 6c ). However, if immunity is ‘infection-dependent’ then the level of protection acquired for subsequent pregnancies could be substantially reduced ( Fig. 6d ). Thus, a better understanding of the mechanisms, by which exposure determines the development of protective immunity, is crucial to understanding the potential for delayed development of pregnancy-associated immunity. Here, we developed a model of the progression of placental malaria, linking the population dynamics of P. falciparum to the results of placental histology at delivery. To our knowledge, this provides the first quantitative estimates of the duration of placental infection, the rate of progression through histologically relevant stages of infection, a quantitative functional form of the acquisition of immunity as a function of exposure in previous pregnancies, and the relationship between the prevalence of placental sequestration and gestational age, parity and transmission intensity. Our results suggest that the observed reductions in prevalence observed in multigravidae are largely attributable to a more rapid clearance of chronic infection, supporting the hypothesis that, following the large inflammatory immune response generated by sequestration during a first pregnancy, the immune system is able to mount a more specific and efficient antibody-led response in subsequent pregnancies [7] . Although there was some evidence that immunity may provide some capability to prevent placental sequestration, which could explain previous experimental findings of women showing ‘perfect immunity’ to ‘artificial innoculation with sporozoites;’, this alone could not reproduce the reduction in chronic infection in higher parity pregnancies observed independently in two data sets [16] , [23] . This faster clearance of chronic infection with increasing parity could be due to increasing titres of antibodies capable of opsonising IEs (which increase with gravidity and have been associated with decreased episodes of parasitaemia, reduced maternal anaemia and antimalarial treatment success [7] , [25] , [26] ). Alternatively, chronic infection might be more rapidly cleared in multigravidae by an increased, but imperfect, anti-CSA-binding antibody response, which limits placental sequestration of IE and facilitates more rapid clearance of placental infection. In contrast, our estimated mean duration of acute infection of around 50 days would seem long enough for an adaptive immune response to develop, but we found no evidence of parity-dependent immunity acting to shorten this duration. It is, however, feasible that enhanced immunity during this stage could contribute to a more rapid clearance of placental infection, even if clearance itself is not achieved before the chronic stage of infection. Ideally, in order to validate our findings, we would assess the extent to which our fitted parameter values replicate the observed patterns in additional data sets. However, to our knowledge the two placental histology data sets used in our analysis are the only sizeable studies in moderate to high transmission settings within the literature in which no pregnancy-specific interventions were being implemented, a consistent histological grading scheme was used, and prevalence and sample size data stratified by gravidity or parity were included. Various studies have found that peripheral parasitaemia early in pregnancy is associated with LBW and anaemia at delivery [27] , [28] , [29] , [30] and it has been suggested that infection at this point in gestation may interfere with placentation and impair the remodelling of spiral arteries to ensure adequate blood flow to the placenta [31] , [32] . Our estimate of a mean duration of active placental infection of around 150 days (that is, 21 weeks) in primigravidae would also appear to suggest that women who develop placental infections early in pregnancy are likely to experience the most prolonged period of placental sequestration. This is because, when infections occur later in pregnancy, they are more likely to be curtailed by the pregnancy reaching term rather than parasite clearance and the high-risk chronic stage may not have developed by delivery. Indeed, we estimated that, regardless of the transmission setting, of the total time primigravidae spend infected during pregnancy, only 30% can be avoided if infection is completely prevented once the placenta becomes susceptible to infection, with the majority of the remaining 70% caused by infections acquired before women become pregnant. Our estimates also suggest that the past stage of infection is very rarely cleared by delivery, suggesting that, in the absence of treatment, the existence of pigment may have good sensitivity as an indicator of previous placental infection and that placental histology is an effective means to determine the proportion of women who have experienced placental malaria at any stage of pregnancy. Our results indicate that many placental infections begin in early pregnancy, shortly after the maternal intervillous spaces become patent and susceptible to sequestration; this finding is conditional on our modelled assumption that any ongoing infection can lead to placental sequestration. Moreover, for multigravidae, our finding that parity-dependent immunity rarely provides sterile protection against an ongoing or incidental infection and instead reduces the time spent with placental infection suggests that the peak in the prevalence of infection in early pregnancy would be even sharper than primigravidae, relative to the prevalence of infection at delivery. This would suggest that, although of paramount importance during first pregnancies, protecting women early and, if possible, immediately before pregnancy should be a priority in all parities. If, as assumed in this analysis, susceptibility to placental infection most commonly begins around the end of the third month of pregnancy, in moderate to high transmission settings, a first placental malaria infection is likely to occur before receipt of the first dose of treatment or prophylaxis under current guidelines for IPTp (4–6 months onwards depending upon the timing of foetal quickening). As the presence of placental infection cannot currently be ascertained during this stage of pregnancy, this assumption is difficult to verify. However, such an effect could explain the peak in peripheral blood infection observed early in the second trimester of pregnancy [17] . Moreover, it would also imply that, while current IPTp strategies may be effective at reducing the duration of time a placenta remains parasitised and thus prevent chronic infection, they are likely to have limited impact on the number of women who experience infection at any stage of pregnancy. Administering preventative therapy at a point of gestation before the placenta becomes susceptible to infection would therefore have the greatest impact on the number of women who experience placental infection. However, timing gestation is difficult before the womb becomes palpable and there are relative contraindications for the provision of SP during the first trimester. Women are also less likely to seek ante-natal care at this stage of pregnancy. Nevertheless, this finding demonstrates the importance of achieving high coverage of an early first dose of preventative therapy, as late dosing is likely to allow sequestration to persist for many weeks before clearance, and highlights the potential benefits of IPTp regimens with drugs, which can be used safely in the first trimester such as chloroquine or choloroquine-azithromycin combinations [33] . Aside from IPTp, this result would also appear to agree with the finding that increases in bednet coverage among women of child-bearing age, by reducing the prevalence of infection before pregnancy, can also have a major impact upon the burden of MiP [34] , [35] . Equally, this finding has obvious implications for the incremental value of any forthcoming vaccine against pregnancy-associated malaria parasites, suggesting that, to optimally protect pregnant women, a vaccine should elicit protective immunity before pregnancy to have maximal impact. The effect that IPTp could have in delaying the acquisition of parity-dependent immunity depends on the assumption made about how exposure to MiP results in protective immunity. Here, we tested two different mechanisms—one assuming that each new infection boosted the level of immunity and the other assuming each infected pregnancy boosted the level of immunity. Both of these mechanisms fitted the data equally well. However, the finding that women receiving IPTp had significantly lower levels of antibody with specificity for pregnancy-associated parasites during a trial in Kenya provides some evidence against the latter mechanism [36] . In reality, as well as known modifiers such as HIV infection [37] , there are many other factors that could influence the level of acquired immunity including the duration of infection, the stage of infection and the time between pregnancies. However, the importance of such factors can only be assessed if detailed data on the individual birth and treatment histories associated with each histology result are analysed. More accurate measures for diagnosis of placental malaria in vivo , such as serum biomarkers of sequestration, or improved placental imaging, could significantly improve our understanding of the processes involved in placental infection, and allow further validation of the model we have proposed. There may also be factors that affect the level of exposure to infection women experience during pregnancy relative to non-pregnant women, such as differences in time spent outdoors or even mosquito biting preferences [38] .. Moreover, there are likely to be seasonal differences in transmission that would not be captured in our model. In the absence of individual-level data on the time of year in which the women deliver, it is difficult to assess the extent to which this has affected our results. However, if the prevalence-level peak in the incidence of placental infection holds true in seasonal settings, then our results would seem to agree with the suggestion that pregnant women at the beginning of a dry season are still relatively vulnerable to the effects of a placental infection owing to the likelihood of an ongoing infection acquired during the rainy season [35] . To more accurately measure the burden of placental infection we still need to define the relationship between the infection and the risk of adverse consequences including LBW. Using our current model estimates, further work is now being undertaken to attempt to quantify this particular risk in terms of the duration, stage (acute, chronic or past) and timing of infection. However, this still will not take into account other aspects of the burden of MiP such as the risk of anaemia, pre-term delivery and the effects of HIV co-infection, all of which would require a large sample of more detailed individual-level data linked to placental histology. For example, the overall effectiveness of IPTp will depend on the effectiveness of clearance and duration of prophylaxis provided. These effects need to be specified both in terms of their impact on observed parasitaemia and on the level of accumulated pigmentation. Histology data For our analysis we required studies that fulfilled the following criteria: (i) histology was conducted on the placentas of a randomly selected cohort of women; (ii) the women received no recorded intervention during pregnancy; (iii) the data were stratified by parity/gravidity; (iv) a contemporary estimate of EIR exists for the setting; (v) a consistent histological categorization across studies. Two studies were retrieved: a study based in Ifakara Town, Tanzania during 1995 (ref. 23 ), where the EIR was estimated to be ∼ 365 infectious bites per-person per year (ibppy) [39] , and a study based in Kilifi District, Kenya during 1996–97 (ref. 16 ), where the EIR was estimated to be 1.5–8 ibppy [40] . There were 1,179 women who had live births for whom placental histology results were available from the Ifakara Town data and 815 from Kilifi District. Although neither study reported women receiving any ongoing intervention, there had been a randomized controlled trial of insecticide-treated-nets in Kilifi District. However, this study found no significant difference between those receiving a bednet and those who did not, either in terms of peripheral or placental parasitaemia or the prevalence of severe anaemia or febrile illness, this study was still included in the analysis [41] . Both used the histological classification described by Ismail et al . [23] This involves four categorizations: not infected (no evidence of parasites or pigment), acute infection (the presence of parasites and no or minimal pigment in fibrin or in cells within fibrin), chronic infection (the presence of parasites and substantial pigmentation) and past infection (absence of parasites and presence of pigment). Both data sets rely upon self-reported fertility data in the form of gravidity (the number of times a women has been pregnant) rather than parity (the number of viable births) and there was not sufficient data to incorporate birth outcome or gestational age at delivery. As a result, we were forced to make the simplifying assumption that gravidity is equivalent to parity and a constant gestational period of 40 weeks. Mathematical model Modelling the results of placental histology at delivery for each setting required linking three distinct sub-models. First, a model of fertility to replicate the age- and parity-dependent patterns of childbirth. Then, for a given pregnancy, the age of the pregnant woman was entered into an age-dependent model of the dynamics of P. falciparum to generate the infection status of the woman at the beginning of the pregnancy and the exposure to infection experienced throughout gestation. This information was then used in a model of placental infection, which also uses a measure of the exposure to infection during any preceding pregnancies to simulate progression through the stages of placental infection (as determined by the histological categorization used) to generate the result of placental histology at delivery. Calculating pregnancy rates Data on pregnancy rates were obtained from the country-specific DHS survey conducted closest in time to the collection of data in each study (Kenya 1998 and Tanzania 1996). Pregnancy rates stratified by 5-year age intervals and parity were calculated by dividing the total number of pregnancies in the 36 months before interview by the women-years of exposure. These age- and parity-dependent rates were then used to generate the age at which a simulated woman becomes pregnant. To ensure the modelled fertility patterns were representative of those within each study area, the data were further sub-divided into rural and urban rates, and the proportion of individuals with birth histories drawn according to each of these sets of rates was chosen to ensure the proportion of multigravidae and primigravidae generated by the fertility model matched the observed proportion within each data set. Model of P. falciparum malaria in general population Full details of the model structure and parameter values are given in Supplementary Note 1 . In brief, the model is an age-structured deterministic model of P. falciparum malaria, which incorporates the following disease stages: susceptible, clinical disease, treatment of clinical disease, prophylaxis, patent infection and sub-patent infection [42] . Immunity develops as a function of both age and exposure to infection. Heterogeneity in the rate at which members of the population are bitten is incorporated by further subdividing the population into five-risk categories. The model was previously fitted to data on microscopy or PCR parasite prevalence by age from 34 locations across Africa and clinical disease data from two sites in Senegal [43] with clinical disease data from a further 18 locations incorporated into the general model fitting in this analysis. The progression of placental infection in primigravidae A large majority of women with detectable peripheral parasitaemia have histological evidence of placental infection [22] and, within the data, the proportion of primigravidae who had some evidence of placental infection was very high (in Ifakara 85% had some evidence of infection). In view of this, and in the interest of model parsimony, we made the baseline assumption that any infection has the potential to sequester within the placenta during first pregnancies and that the minority of peripheral infection at delivery, which are not detected by histology, are the result of recent infection that has yet to sequester. We then conducted a supplementary analysis where we tested the sensitivity of the model to this assumption by fitting scenarios where only 90, 75 or 50% of infections have the ability to sequester (see Supplementary Note 3 ). In the model, maternal blood is assumed to flow into the placenta from the end of the 12th week of gestation. Subsequently, in the absence of any sequestration-blocking immunity and provided infection is sustained for a sufficient duration of time (in our baseline model this was assumed to be 1 week with additional sensitivity analyses conducted using durations of 0, 2 and 3 weeks (see Supplementary Note 4 ), any incidental or ongoing infections result in placental sequestration and an acute stage infection (that is, placental infection where substantial pigment has yet to develop) begins. Each individual infection then progresses through each of the four histological categories of infection according to progression parameters γ A , γ C and γ P ( Fig. 1a ). The mean duration of time spent in each stage of infection is given by the reciprocal of these rates. In the event, a primigravid woman is infected n >1 times, this leads to n independent, and potentially coincident, infections which all progress according to the same parameters. However, the effect of repeated infections on placental histology still needs to be determined. Although, according to the definition of Ismail et al . [23] , any ongoing chronic infection would have sufficient pigment to ensure that the overall classification remained ‘chronic’, the classification arising from the co-existence of an acute infection and remaining pigmentation from a previous infection needs to be defined and will depend upon whether the level of pigmentation is ‘significant’. This was incorporated into the model with a further parameter, ρ , namely the probability a past infection leaves behind ‘significant’ pigmentation ( Fig. 1b ). Incorporating parity-dependent immunity Parity-dependent immunity was incorporated into the model as a function of exposure to placental infections experienced in previous pregnancies. To do this, two distinct types of immunity were explored: Sequestration-blocking immunity whereby the probability that, following infection, the placenta becomes infected, P , decreases with exposure x according to: where v and ξ are parameters. Faster clearance of infection whereby infections progress through the stages of infection at a faster rate. For faster clearance of acute stage infection the clearance rate γ A is assumed to depend on exposure, x , as the function: where τ A , ψ Α and π Α are parameters. Faster clearance of both chronic and past infection, with associated rate parameters, τ c and τ P , power parameters, ψ C and ψ P , and offset parameters π C and π P , were also explored, as well as all possible combinations of the different forms of immunity. Furthermore, two assumptions about the measure of exposure in previous pregnancies, were investigated, with x in the above expressions either representing the total number of infections involved in all sequestration during previous pregnancies, referred to as ‘infection-dependent’ immunity, or the total number of pregnancies in which sequestration occurred (so that x can only increase in increments of 1 following each pregnancy), referred to as ‘infected-pregnancy-dependent’ immunity. Model fitting and comparison Given an underlying prevalence of acute, chronic and past infection, and , within the i th parity category, the probability of observing the number of acute, chronic and past infections ( , and , respectively) from a sample size N i can be calculated using a multinomial distribution Working within a Bayesian framework, the likelihood of any set of model parameters θ given the observed data is then To fit our models of placental infection, the parameters of the general population model were fixed to estimates obtained from the previous fitting and only transmission intensity, defined by the EIR in each setting, was allowed to vary. As both transmission sites were within areas of perennial transmission, it was assumed that the dynamics of P. falciparum infection in the general population could be approximated by the equilibrium state of a model assuming a constant EIR over time. Information about the range of EIR estimates for each transmission setting within the existing literature were incorporated into the fitting procedure using site-specific informative prior distibutions and reasonably uniformative prior distributions were used for all other model parameters. The joint posterior distribution of θ was then estimated using Monte Carlo Markov Chain methods (see Supplementary Note 2 ). The fit of the model to the data for each assumption about parity-dependent immunity was then assessed and compared using the deviance information criterion [44] . Incorporating preventative therapy The potential effect of preventative therapy was investigated by simulating the dynamics of placental sequestration for a synthetic cohort of 200,000 women using 1,000 randomly selected draws from the joint posterior of the final fitted model. The intervention was assumed to result in the immediate clearance of any ongoing parasitaemia, followed by a period of prophylaxis. During this analysis, we only consider the effect of the intervention upon active (acute or chronic) infection in order to avoid the uncertainty about the effect of treatment upon existing pigmentation. How to cite this article: Walker, P.G.T. et al . A model of parity-dependent immunity to placental malaria. Nat. Commun. 4:1609 doi: 10.1038/ncomms2605 (2013).